The evolution of cichlid fish egg-spots is linked with acis-regulatory change The origin of novel phenotypic characters is a key component in organismal diversification; yet, the mechanisms underlying the emergence of such evolutionary novelties are largely unknown. Here we examine the origin of egg-spots, an evolutionary innovation of the most species-rich group of cichlids, the haplochromines, where these conspicuous male fin colour markings are involved in mating. Applying a combination of RNAseq, comparative genomics and functional experiments, we identify two novel pigmentation genes, fhl2a and fhl2b , and show that especially the more rapidly evolving b-paralog is associated with egg-spot formation. We further find that egg-spot bearing haplochromines, but not other cichlids, feature a transposable element in the cis -regulatory region of fhl2b . Using transgenic zebrafish, we finally demonstrate that this region shows specific enhancer activities in iridophores, a type of pigment cells found in egg-spots, suggesting that a cis -regulatory change is causally linked to the gain of expression in egg-spot bearing haplochromines. The de novo evolution of complex phenotypic traits poses a challenge to evolutionary biology [1] , [2] , [3] , [4] , [5] . While selection explains adaptation and speciation in an adequate manner [6] , it is more difficult to conceive how selection would trigger the origin of evolutionary novelties such as insect wings, feathers, tetrapod limbs, flowers, the mammalian placenta, beetle horns or butterfly eye-spots [1] , [4] , [5] , [7] , [8] . The emergence of evolutionary innovations, that is, lineage-restricted traits linked to qualitatively new functions, involves the origin of new developmental modules that are responsible for the identity of these novel characters [4] , [5] . Most of the available evidence suggests that new developmental programs emerge largely through co-option of pre-existing regulatory gene networks via changes in their regulation and deployment (‘old genes playing new tricks’ [5] ). Uncovering the mechanisms of how these developmental modules are co-opted or newly evolved is one of the primary goals of evo-devo research [2] , [3] , [5] , [7] , [8] . Anal fin egg-spots are an evolutionary innovation in the so-called ‘haplochromines’ [9] ( Fig. 1a and Supplementary Fig. 1 ), the most species-rich group of cichlid fishes, best known for their spectacular adaptive radiations in the East African lakes Victoria and Malawi [10] , [11] . Adult males of ~1,500 cichlid species feature this pigmentation trait in the form of conspicuously coloured circular markings [9] , [11] , [12] . Haplochromine egg-spots vary substantially in colour, shape, number and arrangement between species ( Fig. 1b ), and even within species a certain degree of variation is observed. In some species, also females show egg-spots, which are then much less pronounced and colourful. The function of egg-spots has been implicated with the mating behaviour of the female-mouthbrooding haplochromines [12] , [13] . Immediately upon spawning, a haplochromine female gathers up her eggs into the mouth; the male then presents his egg-spots to which the female responds by snatching and bringing her mouth close to the male’s genital opening; upon discharging sperm, the eggs become fertilized inside the female’s mouth ( Fig. 1c ). The mother subsequently broods and carries her progeny in the oral cavities for several weeks after fertilization. 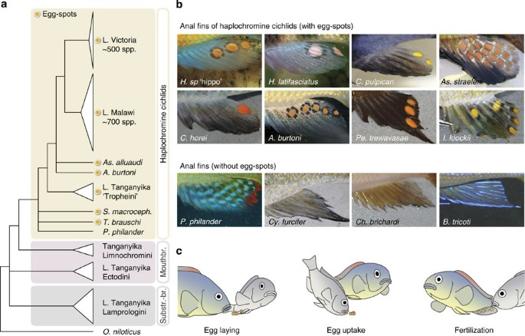Figure 1: The egg-spots of haplochromine cichlids. (a) Phylogeny of the East African cichlid fishes based on a new multimarker data set. The haplochromines are the most species-rich and derived group of cichlids in East Africa. One of the common features of haplochromines is the presence of egg-spots on the anal fin of males. Note that one of the ancestral lineages, represented here byP. philander, does not show this characteristic trait9,33. Substr-br, substrate brooders; mouthbr, mouthbrooders; spp.: species. (b) Examples of male anal fin patterns in East African cichlids. Haplochromine egg-spots (upper panel) vary in size, shape, number and colouration. Non-haplochromines and basal haplochromineP. philander(lower panel) do not show this trait. (c) A typical mating cycle of haplochromine cichlids. Figure 1: The egg-spots of haplochromine cichlids. ( a ) Phylogeny of the East African cichlid fishes based on a new multimarker data set. The haplochromines are the most species-rich and derived group of cichlids in East Africa. One of the common features of haplochromines is the presence of egg-spots on the anal fin of males. Note that one of the ancestral lineages, represented here by P. philander , does not show this characteristic trait [9] , [33] . Substr-br, substrate brooders; mouthbr, mouthbrooders; spp. : species. ( b ) Examples of male anal fin patterns in East African cichlids. Haplochromine egg-spots (upper panel) vary in size, shape, number and colouration. Non-haplochromines and basal haplochromine P. philander (lower panel) do not show this trait. ( c ) A typical mating cycle of haplochromine cichlids. Full size image Here we are interested in the molecular basis of the anal fin egg-spots of haplochromine cichlids. The main advantages of the cichlid egg-spot system are that (i) the evolutionary innovation of interest emerged just a few million years ago and hence is recent compared with most other evolutionary novelties studied so far [9] , [10] , [14] ; (ii) the phylogenetic context in which the novel trait evolved is known and living sister clades to the lineage featuring the novelty still exist [9] , [15] , [16] ; and (iii) the genomes of two outgroup species lacking the trait and of three derived species featuring the trait are available. This allows us to study early events involved in the origin of an evolutionary innovation in an assemblage of phenotypically diverse, yet closely related and genetically similar species [14] . Using RNAseq, we identify two novel candidate pigmentation genes, the a- and b-paralogs of the four and a half LIM domain protein 2 ( fhl2 ) gene, and show that both genes, but especially the more rapidly evolving b-copy, are associated with the formation of egg-spots. We then find that egg-spot bearing haplochromines—but not an egg-spot-less ancestral haplochromine and not the representatives from more basal cichlid lineages—exhibit a transposable element insertion in close proximity to the transcription initiation site of fhl2b . A functional assay with transgenic zebrafish reveals that only a haplochromine-derived genetic construct featuring the SINE (short interspersed repetitive element) insertion drove expression in a special type of pigment cells, iridophores. Together, our data suggest that a cis -regulatory change (probably in the form of a SINE insertion) is responsible for the gain of expression of fhl2b in iridophores, contributing to the evolution of egg-spots in haplochromine cichlids. fhl2 paralogs: novel candidates for egg-spot morphogenesis As a first step, we performed an Illumina-based comparative transcriptomic experiment (RNAseq) between male (with egg-spots) and female (without egg-spots) anal fins in the haplochromine cichlid Astatotilapia burtoni . 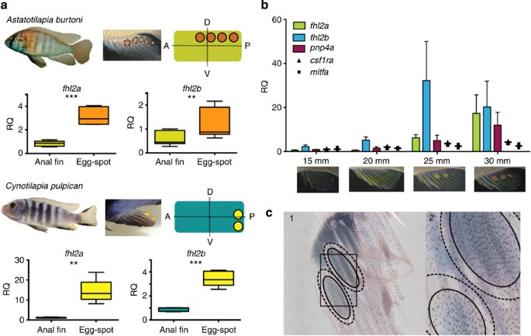Figure 2: The role offhl2aandfhl2bin egg-spot formation. (a) qPCR experiments reveal that both genes are overexpressed in egg-spot compared with adjacent anal fin tissue in the haplochromine cichlidsA. burtoniandC. pulpican(**P<0.01; ***P<0.001; RQ, relative quantity). Images of male fishes of the two species, their anal fins and a scheme showing the distribution of egg-spots are provided. (b) Expression profiles offhl2aandfhl2bduring the ontogenetic development of egg-spots inA. burtoni(note that egg-spots are absent in juveniles and only form when males become sexually mature; see ref.22for further details). The values on thexaxis represent fish standard length in millimetres (three replicates per developmental stage were used). The error bars represent the s.e.m.fhl2bshows the largest increase in expression overall and its expression profile mimics the formation of egg-spots. Three other pigmentation genes (pnp4a, csf1raandmitfa) were included for comparative reasons.csf1raandmitfashow a much smaller increase in gene expression during egg-spot development thanfhl2aand especiallyfhl2b, whilepnp4ashows a constant increase in gene expression throughout the development of egg-spots. (c) RNAin situhybridization experiments revealed that bothfhl2paralogs (results only shown forfhl2b) are primarily expressed in the colourful inner circle of haplochromine egg-spots (defined by the solid line) and not in the transparent outer ring (defined by the dashed line). Expression was also observed in the proximal fin region, which also contains pigment cells. Panel 2 is a close-up from the region defined by the square in panel 1. Two of the most differentially expressed genes according to RNAseq were the a- and b-paralogs of fhl2 (~4 log 2 -fold and ~5 log 2 -fold differences, respectively; see Supplementary Table 2 ). These paralogs result from the teleost genome duplication [17] ( Supplementary Fig. 2 ). The four and a half LIM domain protein 2 (Fhl2) is known as a transcriptional co-activator of the androgen receptor and the Wnt -signalling pathway [18] , [19] ; Fhl2 plays a role in cell-fate determination and pattern formation, in the organization of the cytoskeleton, in cell adhesion, cell motility and signal transduction; furthermore, it regulates the development of heart, bone and musculature in vertebrates [20] , [21] . Expression of fhl2a and fhl2b is egg-spot specific To confirm the results obtained by RNAseq, we performed quantitative real-time PCR (qPCR) experiments ( Fig. 2a ), this time also comparing egg-spot versus non-egg-spot tissue within male anal fins. In addition, we tested another haplochromine species, Cynotilapia pulpican , with a different egg-spot arrangement to exclude positional effects of gene expression on the anal fin. In both species, the two duplicates of fhl2 were overexpressed in egg-spots ( A. burtoni : fhl2a : t 5 =10.77, P =0.0001; fhl2b: t 5 =4.362, P =0.0073; C. pulpican : fhl2a : t 4 =5.031, P =0.0073; fhl2b: t 4 =9.154, P =0.0008). We then tested the expression of both fhl2 paralogs in the four main developmental stages of egg-spot formation in A. burtoni [22] and compared it with other candidate pigmentation genes (including the previously identified xanthophore marker csf1ra , the melanophore marker mitfa and the iridophore marker pnp4a ). We found that the expression of both fhl2 paralogs increases substantially throughout anal fin and egg-spot development, and both genes showed higher expression levels compared with the other pigmentation genes ( Fig. 2b ); fhl2b shows the highest increase in expression exactly when egg-spots begin to form. Furthermore, we corroborate that the expression domain of both fhl2a and fhl2b matches the conspicuously coloured inner circle of egg-spots with RNA in situ hybridization (see Fig. 2c for results on fhl2b ). Figure 2: The role of fhl2a and fhl2b in egg-spot formation. ( a ) qPCR experiments reveal that both genes are overexpressed in egg-spot compared with adjacent anal fin tissue in the haplochromine cichlids A. burtoni and C. pulpican (** P <0.01; *** P <0.001; RQ, relative quantity). Images of male fishes of the two species, their anal fins and a scheme showing the distribution of egg-spots are provided. ( b ) Expression profiles of fhl2a and fhl2b during the ontogenetic development of egg-spots in A. burtoni (note that egg-spots are absent in juveniles and only form when males become sexually mature; see ref. 22 for further details). The values on the x axis represent fish standard length in millimetres (three replicates per developmental stage were used). The error bars represent the s.e.m. fhl2b shows the largest increase in expression overall and its expression profile mimics the formation of egg-spots. Three other pigmentation genes ( pnp4a, csf1ra and mitfa ) were included for comparative reasons. csf1ra and mitfa show a much smaller increase in gene expression during egg-spot development than fhl2a and especially fhl2b , while pnp4a shows a constant increase in gene expression throughout the development of egg-spots. ( c ) RNA in situ hybridization experiments revealed that both fhl2 paralogs (results only shown for fhl2b ) are primarily expressed in the colourful inner circle of haplochromine egg-spots (defined by the solid line) and not in the transparent outer ring (defined by the dashed line). Expression was also observed in the proximal fin region, which also contains pigment cells. Panel 2 is a close-up from the region defined by the square in panel 1. Full size image fhl2a and fhl2b evolved under purifying selection In general, phenotypic differences can arise via mutations affecting the function of proteins or via changes in gene regulation [5] . Therefore, we examined coding sequence evolution in the two fhl2 paralogs to test for positive selection and potential change of function in a phylogenetically representative set of 26 East African cichlids. We found that the two fhl2 genes are highly conserved in cichlids, with few amino-acid differences between species and an average genetic divergence (0.4% in fhl2a and 0.7% in fhl2b ) that lies below the transcriptome-wide average of 0.95% (ref. 23 ). None of the observed amino-acid changes was correlated with the egg-spot phenotype ( Supplementary Table 7 ). Greater functional specialization of fhl2b in haplochromines Usually, after a gene duplication event, the duplicates go through a period of relaxed selection, during which one of the two copies can diversify and acquire new functions [24] . We found that the b-copy of fhl2 shows an elevated rate of molecular evolution compared with its paralog ( fhl2a ), which more closely resembles the ancestral sequence ( Fig. 3a ). An additional series of qPCR experiments in 12 tissues revealed that, in cichlids, fhl2a is primarily expressed in heart, bony structures and muscles, whereas fhl2b is highly expressed in the eye, and further in skin and the egg-spots of haplochromines ( Fig. 3b,c ). This is different to the gene expression profiles in medaka, where both duplicates are highly expressed in heart, skin and eye tissues; and in zebrafish, where the two paralogs are primarily expressed in heart, eye and (pharyngeal) jaw tissues, with fhl2a showing rather low levels of gene expression ( Supplementary Figs 3 and 4 ). When compared with the other teleost fishes examined here, our results suggest that the haplochromine fhl2a retained most of the previously described functions, whereas the more rapidly evolving fhl2b obtained new expression patterns. Together, the gene expression profile and the pattern of sequence evolution make fhl2b a prime candidate gene for the morphogenesis of haplochromine egg-spots. 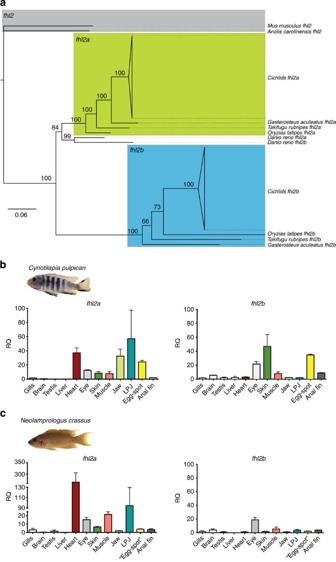Figure 3: Gene tree of the twofhl2paralogs and expression profiling in East African cichlid fishes. (a) Bayesian inference phylogeny of the orthology and paralogy relationships between cichlids, other teleosts (O. latipes,D. rerio, Ta. rubripesandG. aculeatus) and tetrapods (Anolis carolinensisandMus musculus)fhl2sequences. This gene tree is important for generating functional hypotheses about both duplicates, and to infer the ancestral state of thefhl2gene before duplication. Our phylogeny indicates thatfhl2ais more similar to the ancestral state, whilefhl2bis apparently evolving faster in teleosts. Values at the tree nodes represent posterior probabilities. InSupplementary Fig. 2, we present a synteny analysis supporting the origin of teleostfhl2 duplicates in the teleost genome duplication. (b) Relative quantity (RQ) offhl2aandfhl2bgene expression in 12 tissues (three replicates per tissue) inC. pulpican, an egg-spot bearing haplochromine from Lake Malawi. The error bars represent the s.e.m. (c) RQ offhl2aandfhl2bgene expression in 12 tissues inN. crassus, a substrate spawning lamprologine that has no egg-spots. In both species, gill tissue was used as reference; inN. crassus, ‘egg-spots’ corresponds to the fin region where haplochromines would show the egg-spot trait. InC. pulpican(b),fhl2ais highly expressed in heart, in pigmented tissues (eye, skin and egg-spot) and in craniofacial traits (oral jaw and lower pharyngeal jaw);fhl2bis mainly expressed in the pigmented tissues.N. crassus(c) shows a similar expression patterns forfhl2aandfhl2b, with the difference thatfhl2adoes not show high expression levels in jaw tissues, andfhl2bis not highly expressed in skin and fin tissue. These results suggest thatfhl2bshows a higher functional specialization, and that it might be involved in the morphogenesis of sexually dimorphic traits such as pigmented traits including egg-spots. LPJ, lower pharyngeal jaw bone. Figure 3: Gene tree of the two fhl2 paralogs and expression profiling in East African cichlid fishes. ( a ) Bayesian inference phylogeny of the orthology and paralogy relationships between cichlids, other teleosts ( O. latipes , D. rerio, Ta. rubripes and G. aculeatus ) and tetrapods ( Anolis carolinensis and Mus musculus ) fhl2 sequences. This gene tree is important for generating functional hypotheses about both duplicates, and to infer the ancestral state of the fhl2 gene before duplication. Our phylogeny indicates that fhl2a is more similar to the ancestral state, while fhl2b is apparently evolving faster in teleosts. Values at the tree nodes represent posterior probabilities. In Supplementary Fig. 2 , we present a synteny analysis supporting the origin of teleost fhl 2 duplicates in the teleost genome duplication. ( b ) Relative quantity (RQ) of fhl2a and fhl2b gene expression in 12 tissues (three replicates per tissue) in C. pulpican , an egg-spot bearing haplochromine from Lake Malawi. The error bars represent the s.e.m. ( c ) RQ of fhl2a and fhl2b gene expression in 12 tissues in N. crassus , a substrate spawning lamprologine that has no egg-spots. In both species, gill tissue was used as reference; in N. crassus , ‘egg-spots’ corresponds to the fin region where haplochromines would show the egg-spot trait. In C. pulpican ( b ), fhl2a is highly expressed in heart, in pigmented tissues (eye, skin and egg-spot) and in craniofacial traits (oral jaw and lower pharyngeal jaw); fhl2b is mainly expressed in the pigmented tissues. N. crassus ( c ) shows a similar expression patterns for fhl2a and fhl2b , with the difference that fhl2a does not show high expression levels in jaw tissues, and fhl2b is not highly expressed in skin and fin tissue. These results suggest that fhl2b shows a higher functional specialization, and that it might be involved in the morphogenesis of sexually dimorphic traits such as pigmented traits including egg-spots. LPJ, lower pharyngeal jaw bone. Full size image fhl2b shows an AFC-SINE insertion in species with egg-spot Since there were no changes in the coding regions of fhl2a and fhl2b that are specific to the egg-spot bearing haplochromines, we shifted our focus towards the analysis of putative regulatory elements, exploring the recently available genomes of five East African cichlids (including the egg-spot bearing haplochromines A. burtoni , Pu. nyererei , Metriaclima zebra and the egg-spot-less non-haplochromines Neolamprologus brichardi and Oreochromis niloticus ). The non-coding region of fhl2a shows homology with other teleosts ( Oryzias latipes , Takifugu rubripes , Tetraodon nigroviridis and Gasterosteus aculeatus ) and we identified four conserved non-coding elements (CNEs) in all species examined ( Supplementary Fig. 5a ). These CNEs might thus represent conserved regulatory regions responsible for ancestral conserved functions of fhl2a in teleosts. We might be missing cichlid-specific regulatory regions in important upstream regions although, as our capacity to detect lineage-specific enhancers is limited owing to the small sample size for each lineage and the high background conservation level present in cichlids. Concerning fhl2b , we did not find any CNE that is shared by cichlids and other teleosts ( Supplementary Fig. 5b ). Strikingly, however, we found a major difference that is shared by the three egg-spot bearing haplochromines: the presence of a transposable element upstream of fhl2b . Specifically, we identified a SINE belonging to the cichlid-specific AFC-SINEs (African cichlid family of SINEs [25] ), which inserted ~800-bp upstream of the transcriptional start site of fhl2b ( Supplementary Fig. 6 ). To confirm that this insertion is associated with the egg-spot phenotype, we sequenced the upstream region of fhl2b in 19 cichlid species. The insertion was indeed present in nine additional, egg-spot bearing haplochromine species, yet absent in all 10 non-haplochromines examined ( Supplementary Table 8 ). Importantly, we found that one haplochromine species lacks the AFC-SINE element, namely P. philander. This species belongs to one of the basal lineage of haplochromines ( Fig. 1a ), which is characterized by the absence of egg-spots ( Fig. 1b ). This suggests that the AFC-SINE upstream of fhl2b is not characteristic to the entire haplochromine clade, but to those that feature egg-spots, thus linking the SINE insertion to the origin of this evolutionary innovation. Haplochromine fhl2b regulatory region drives iridophore expression A long-standing hypothesis proposes that ubiquitous genomic repeat elements are potential regulators of transcription, and could thereby generate evolutionary variations and novelties [26] , [27] . SINEs are known for their capability of ‘transcriptional rewiring’, that is, to change the expression patterns of genes by bringing along new regulatory sequences when inserted in close proximity to a gene’s transcriptional initiation site [7] , [28] . In order to test whether the insertion of an AFC-SINE close to fhl2b functions as an enhancer of gene expression, we aimed for a functional experiment. We were particularly interested to find out whether there were changes in enhancer activity between AFC-SINE-positive haplochromines and other cichlids lacking both the insertion and the egg-spot phenotype. To this end, we designed reporter constructs containing the upstream region of fhl2b (~2 kb upstream to intron 1) of three cichlid species linked to the coding region of green fluorescent protein (GFP), and injected these constructs into zebrafish ( Danio rerio ) embryos to generate transgenic lines. We switched to the zebrafish system here, as no functioning transgenesis was available for haplochromine cichlids at the time the study was performed (owing to the small number of eggs per clutch associated with the characteristic female-mouthbrooding behaviour). The three constructs were derived from A. burtoni (haplochromine with egg-spots, AFC-SINE + ), P. philander (haplochromine without egg-spots, AFC-SINE − ) and N. sexfasciatus (lamprologine, AFC-SINE − ), respectively ( Fig. 4a ). 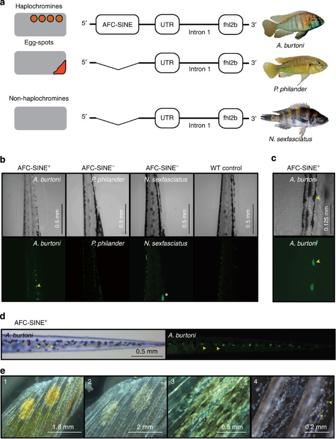Figure 4: The molecular basis of egg-spot formation. (a) The egg-spot bearing haplochromines feature an AFC-SINE insertion in close proximity to the transcriptional start site offhl2b, which is absent in the ancestral and egg-spot-less genusPseudocrenilabrusand in all non-haplochromines. The sequences from the three species shown here were the ones used to engineer the reporter constructs, where thefhl2bcoding sequence was substituted by GFP. (b) In transgenic zebrafish, only the AFC-SINE+construct showed GFP expression in the iridophores, a type of pigment cells (one of them is indicated by a yellow arrow). The upper panel depicts bright-field images of 3-day-old zebrafish embryo trunks; the lower panel shows the respective embryos under ultraviolet light. The green signal in the AFC-SINE negativeN. sexfasciatusline (marked with an asterisk) is auto-fluorescence from the yolk extension. (c) Higher magnification image fromA. burtoniAFC-SINE+reporter construct driving GFP expression in the iridophores. Orientation inb,c: bottom: anterior, top: posterior. (d) Top-down view of a trunk of a 3-day-old AFC-SINE-positive zebrafish embryo. The left panel depicts a bright-field image where the iridophores of the dorsal stripe are illuminated by the incident light (yellow arrows). The right panel depicts GFP expression of the same embryo. The GFP signal co-localizes with iridophores. (e) Cellular basis of egg-spots: this series of images shows that egg-spots are made up of xanthophores, iridophores and scattered melanophores. Image 1 shows anA. burtonifin with two egg-spots. Image 2 shows the same fin without pteridine pigments (xanthophores are not visible anymore). Images 3 and 4 are higher magnification images of the egg-spots without pteridine under slightly different light conditions confirming that egg-spots have a high density of iridophores (examples of this cell type are highlighted with arrows). UTR, untranslated region. Figure 4: The molecular basis of egg-spot formation. ( a ) The egg-spot bearing haplochromines feature an AFC-SINE insertion in close proximity to the transcriptional start site of fhl2b , which is absent in the ancestral and egg-spot-less genus Pseudocrenilabrus and in all non-haplochromines. The sequences from the three species shown here were the ones used to engineer the reporter constructs, where the fhl2b coding sequence was substituted by GFP. ( b ) In transgenic zebrafish, only the AFC-SINE + construct showed GFP expression in the iridophores, a type of pigment cells (one of them is indicated by a yellow arrow). The upper panel depicts bright-field images of 3-day-old zebrafish embryo trunks; the lower panel shows the respective embryos under ultraviolet light. The green signal in the AFC-SINE negative N. sexfasciatus line (marked with an asterisk) is auto-fluorescence from the yolk extension. ( c ) Higher magnification image from A. burtoni AFC-SINE + reporter construct driving GFP expression in the iridophores. Orientation in b , c : bottom: anterior, top: posterior. ( d ) Top-down view of a trunk of a 3-day-old AFC-SINE-positive zebrafish embryo. The left panel depicts a bright-field image where the iridophores of the dorsal stripe are illuminated by the incident light (yellow arrows). The right panel depicts GFP expression of the same embryo. The GFP signal co-localizes with iridophores. ( e ) Cellular basis of egg-spots: this series of images shows that egg-spots are made up of xanthophores, iridophores and scattered melanophores. Image 1 shows an A. burtoni fin with two egg-spots. Image 2 shows the same fin without pteridine pigments (xanthophores are not visible anymore). Images 3 and 4 are higher magnification images of the egg-spots without pteridine under slightly different light conditions confirming that egg-spots have a high density of iridophores (examples of this cell type are highlighted with arrows). UTR, untranslated region. Full size image We were able to produce stable transgenic zebrafish lines for each of the three constructs to examine the expression of GFP. Importantly, we found striking differences in expression between the A. burtoni construct and the two constructs lacking the AFC-SINE. Of the three reporter lines, only the AFC-SINE + showed GFP expression in iridophores, a silvery-reflective type of pigment cells ( Fig. 4b,c and Supplementary Fig. 7 ). This experiment demonstrates the presence of novel enhancer activities in the regulatory region of fhl2b in derived haplochromines and strongly suggests that these came along with the SINE insertion. Iridophores and egg-spot development The egg-spot phenotype has previously been associated with pigment cells containing pteridines (xanthophores) [16] , [22] , whereas our new results indicate an auxiliary role of iridophores in egg-spot formation. We thus re-evaluated the adult egg-spot phenotype by removing the pteridine pigments of the xanthophores ( Fig. 4e ). We indeed found that A. burtoni egg-spots show a high density of iridophores, which is further corroborated by the increase in gene expression of the iridophore marker pnp4a during egg-spot formation ( Fig. 2b ). With the exception of the proximal region of the anal fin, the number of iridophores is greatly reduced in the fin tissue surrounding egg-spots ( Supplementary Fig. 8a ). Interestingly, this proximal region is the only area of the anal fin besides the egg-spots where we observed fhl2 expression with RNA in situ hybridization (see Fig. 2c for fhl2b ), once more linking fhl2 expression with iridophores (and less so with xanthophores, which are very rare in this region). In the non-haplochromine N. crassus , which features a yellow anal fin pattern containing xanthophores, we did not find iridophores in the xanthophore-rich region ( Supplementary Fig. 9 ), suggesting that the xanthophore/iridophore pattern is unique to haplochromine egg-spots. Importantly, we also observed that iridophores appear early in the newly forming egg-spot of haplochromines, that is, before the first xanthophores start to aggregate ( Supplementary Fig. 8b ). In zebrafish, stripe development is initiated by iridophores, which serve as morphological landmarks for stripe orientation in that they attract further pigment cells such as xanthophores by expressing the csf1 ligand gene [29] , [30] . Interestingly, it has previously been shown that a gene encoding a Csf1 receptor known for its role in xanthophore development in zebrafish, csf1ra , is expressed in haplochromine egg-spots [16] . We thus examined the expression of the ligand csf1b and show that its relative level of gene expression doubles during egg-spot development, and that this increase coincides with the emergence of the phenotype ( Supplementary Fig. 10 ). This leads us to suggest that a similar pigment cell type interaction mechanism might be involved in egg-spot patterning as the one described for zebrafish [29] , [30] . The specific mode of action of fin patterning in haplochromine cichlids, and how Fhl2b interacts with the Csf1/Csf1r system, remains to be studied in the future. Contribution of fhl2a in egg-spot formation The role of the more conserved and functionally constrained a-paralog of fhl2 in egg-spot development cannot be dismissed. Its temporally shifted increase in gene expression compared with fhl2b ( Fig. 2b ) suggests that fhl2a most likely acts as a more downstream factor involved in pigment pattern formation. We were nevertheless interested in uncovering the regulatory region responsive for this expression pattern. The first intron of fhl2a shows two CNEs that are common across percomorph fish ( Supplementary Fig. 5 ). Using the same strategy as described above, we generated a transgenic zebrafish line containing exon 1 and intron 1 of A. burtoni linked to GFP. This construct drove expression in heart in zebrafish embryos, which is consistent with the reported function of fhl2a in tetrapods [20] , whereas there was no indication of a pigment cell related function for this reporter construct ( Supplementary Fig. 7e ). An alignment between the genomic regions of the two fhl2 paralogs shows that there were no CNEs in common and generally very little homology between them, suggesting that the regulation of the expression of fhl2a in egg-spots might proceed in a different way ( Supplementary Fig. 11 ). In this study, we were interested in the genetic and developmental basis of egg-spots, an evolutionary innovation of the most species-rich group of cichlids, the haplochromines, where these conspicuous colour markings on the anal fins of males play an important role in mating [11] , [12] , [13] ( Fig. 1 ). We first performed a comparative RNAseq experiment that led to the identification of two novel candidate pigmentation genes, the a- and b-paralogs of the four and a half LIM domain protein 2 ( fhl2 ) gene. We then confirmed, with qPCR and RNA in situ hybridization, that the expression domain of both duplicates indeed matches the conspicuously coloured inner circle of egg-spots ( Fig. 2 ). Especially the more rapidly evolving b-copy of fhl2 emerged as strong candidate gene for egg-spot development, as its expression profile mimics the formation of egg-spots ( Figs 2b and 3 ). Interestingly, we found that the egg-spot bearing haplochromines, but not other cichlids, feature a transposable element in the cis -regulatory region of fhl2b . Finally, making use of transgenic zebrafish, we could show that a cis -regulatory change in fhl2b in the ancestor of the egg-spot bearing haplochromine cichlids (most likely in the form of the AFC-SINE insertion) resulted in a gain of expression in iridophores, a special type of pigment cells found in egg-spots ( Fig. 4 ). This in turn might have led to changes in iridophore cell behaviour and to novel interactions with pigmentation genes ( csf1b , csf1ra and pnp4a ), thereby contributing to the formation of egg-spots on male anal fins. The specific mode of action of the SINE insertion, and how the fhl2b locus interacts with these other pigmentation genes remains elusive at present. Addressing these questions would require functional studies in haplochromines, which are, however, hampered by the specific mechanisms involved in the trait complex of interest (mouthbrooding makes it notoriously difficult to obtain enough eggs—in a controlled manner—to make such experiments feasible). Our results are also suggestive of an important role of the a-copy of fhl2 in cichlid evolution. With our qPCR experiments, we provide strong evidence that fhl2a is involved in jaw tissue in zebrafish ( Supplementary Fig. 3 ) and, importantly, in the pharyngeal jaw apparatus of cichlids ( Fig. 3b,c ), another putative evolutionary innovation of this group. The pharyngeal jaw apparatus is a second set of jaws in the pharynx of cichlids that is functionally decoupled from the oral jaws and primarily used to process food [11] , [12] , [15] . Interestingly, fhl2a has previously been implicated in the evolution of fleshy lips in cichlids [31] , which is yet another ecologically relevant trait. From a developmental perspective, the main tissues underlying these traits—the cranio-facial cartilage (the jaw apparatus) and pigment cells (egg- spots)—have the same origin, the neural crest, which itself is considered an evolutionary key innovation of vertebrates [32] . It thus seems that the function of fhl2 in cichlids may have been split into (a) an ecologically important, that is, naturally selected, scope of duties, and (b) a role in colouration and pigmentation more likely to be targeted by sexual selection. Taken together, our study permits us to propose the following hypothesis for the origin of cichlid egg-spots: In one of the early, already female-mouthbrooding, haplochromines the insertion of a transposable element of the AFC-SINE family in the cis -regulatory region of fhl2b , and its associated recruitment to the iridophore pigment cell pathway, mediated the evolution of egg-spots on the anal fins—possibly from the so-called perfleckmuster common to many cichlids [16] . The conspicuous anal fin spots were fancied by haplochromine females, which—just like many other cichlids and also the ancestral and egg-spot-less haplochromine genus Pseudocrenilabrus —have an innate bias for yellow/orange/red spots that resemble carotenoid-rich prey items [33] , leading to the fixation of the novel trait. In today’s haplochromines, egg-spots seem to have a much broader range of functions related to sexual selection [34] . Most of the currently studied evolutionary innovations comprise relatively ancient traits (for example, flowers, feathers, tetrapod limb, insect wings and mammalian placenta), thereby making it difficult to scrutinize their genetic and developmental basis. Here we explored a recently evolved novelty, the anal fin egg-spots of male haplochromine cichlids. We uncovered a regulatory change in close proximity to the transcriptional start site of a novel iridophore gene that likely contributes to the molecular basis of the origin of egg-spots in the most rapidly diversifying clade of vertebrates. This, once more, illustrates the importance of changes in cis -regulatory regions in morphological evolution [2] . Samples Laboratory strains of A. burtoni , C. pulpican , Astatoreochromis alluaudi , Pu. nyererei , Labidochromis caeruleus , Pseudotropheus elegans and N. crassus were kept at the University of Basel (Switzerland) under standard conditions (12 h light/12 h dark; 26 °C, pH 7). Before dissection, all specimens were euthanized with MS 222 (Sigma-Aldrich, USA) following an approved procedure (permit no. 2317 issued by the cantonal veterinary office Basel). Individuals of all other specimens were collected in the southern region of Lake Tanganyika (Zambia) under the permission of the Lake Tanganyika Unit, Department of Fisheries, Republic of Zambia, and processed in the field following our standard operating procedure [15] . Tissues for RNA extraction were stored in RNAlater (Ambion, USA), and tissues for genomic DNA extraction were stored in ethanol and shipped to the University of Basel. RNA and DNA extractions Isolation of RNA was performed according to the TRIzol protocol (Invitrogen, USA) after incubating the dissected tissues in 750 μl of TRIzol at 4 °C overnight or, alternatively, for 8–16 h (in order to increase the RNA yield after long-term storage). The tissues were then homogenized with a BeadBeater (FastPrep-24; MP Biomedicals, France). Subsequent DNase treatment was performed with DNA-Free kit (Ambion). RNA quantity and quality was determined with a NanoDrop 1000 spectrophotometer (Thermo Scientific, USA). cDNA was produced using the High Capacity RNA-to-cDNA kit (Applied Biosystems, USA). Genomic DNA was extracted using a high salt extraction method (modified from ref. 35 ). Phylogenetic analyses DNA extraction of 18 specimens of East African cichlid fishes was conducted as described above. For the amplification of nine nuclear markers ( rag , gapdhs , s7 , bmp4 , ednrb1 , mitfa , tyr , hag and csfr1 ), we used the primer sets published in ref. 36 . The sequences of M. zebra, O. niloticus and N. brichardi were extracted from the respective genome assemblies ( http://www.broadinstitute.org/models/tilapia ). The data for Astatoreochromis alluaudi, Thoracochromis brauschi and Serranochromis macrocephalus were collected with Sanger sequencing following the method described in ref. 36 , all other data were generated by amplicon sequencing with 454 GS FLX system at Microsynth, Switzerland, following the manufacturer’s protocols [37] , [38] . Sequences were quality filtered using PRINSEQ (length: 150 bp minimum; low quality: mean ≥15; read duplicates) [39] and assembled with Burrows-Wheeler Aligner, Smith-Waterman alignment (BWA-SW) followed by visual inspection and consensus sequence generation in Geneious 6.1.6 (ref. 40 ). As a tenth marker, we included mitochondrial NADH dehydrogenase subunit 2 (ND2) sequences available on GenBank (see Supplementary Table 1 for accession numbers). Since the ednrb1 gene sequence is not available in the N. brichardi genome assembly, we used the gene sequence from its sister species, N. pulcher , instead. Sequences were aligned with MAFFT [41] and the most appropriate substitution model of molecular evolution for each marker was determined with JMODELTEST v2.1.3 (ref. 42 ) and BIC [43] . The partitioned data set (5,051 bp) was then subjected to phylogenetic analyses in MRBAYES v3.2.1 (ref. 44 ) and GARLI v2.0 (ref. 45 ). MRBAYES was run for 10,000,000 generations with two runs and four chains in parallel and a burn-in of 25%, GARLI was run 50 times followed by a bootstrap analysis with 500 replicates. SUMTREES v3.3.1 of the DENDROPY package v3.12.0 (ref. 46 ) was used to summarize over the replicates and to map bootstrap values to the ML topology. Differential gene expression analysis using RNAseq We used a transcriptomic approach (RNAseq) to identify genes differentially expressed between male and female anal fins of A. burtoni . Library construction and sequencing of RNA extracted from three male and three female anal fins (at the developmental stage of 30 mm; Fig. 2 ) was performed at the Department of Biosystems Science and Engineering, University of Basel and ETH Zurich. The samples were sequenced on an Illumina Genome Analyzer IIx. Each sample was sequenced in one lane and with a read length of 76 bp. The reads were then aligned to an embryonic A. burtoni reference transcriptome assembled by Broad Institute ( http://www.broadinstitute.org/models/tilapia ). This transcriptome is not annotated and each transcript has a nomenclature where the first term codes for the parent contig and the third term codes for alternatively spliced transcripts (CompX_cX_seqX). The reference transcriptome was indexed using NOVOINDEX ( www.novocraft.com ) with default parameters. Using NOVOALIGN ( www.novocraft.com ), the RNAseq reads were mapped against the reference transcriptome with a maximum alignment ( t ) score of 30, a minimum of good-quality base pair per read (l) of 25 and a successive trimming factor (s) of 5. Reads that did not match these criteria were discarded. Since the reference transcriptome has multiple transcripts/isoforms belonging to the same gene, all read alignment locations were reported (rALL). The mapping results were reported (o) in SAM format. The output SAM file was then transformed into BAM format, sorted, indexed and converted to count files (number of reads per transcript) using SAMTOOLS version 0.1.18 (ref. 47 ). The count files were subsequently concatenated into a single data set—count table—and analysed with the R package EDGER [48] in order to test for significant differences in gene expression between male and female anal fins. The 10 most differentially expressed transcripts were identified by BLASTx [49] against GenBank’s non-redundant database ( Supplementary Table 2 ). We selected two genes out of this list for in-depth analyses— fhl2a and fhl2b —for the following three reasons: (i) fhl2b was the gene showing the highest difference in expression between male and female anal fins; (ii) the difference in gene expression in its paralog, fhl2a , was also significantly high; and (iii) the functional repertoire of the Fhl2 protein family indicates that these might be strong candidates for the morphogenesis of a secondary male colour trait. Differential gene expression analysis using qPCR The expression patterns of fhl2a and fhl2b were further characterized by means of qPCR in three species, A. burtoni , C. pulpican and N. crassus . The comparative cycle threshold method [50] was used to calculate differences in expression between the different samples using the ribosomal protein L7 ( rpl7 ) and the ribosomal protein SA3 ( rpsa3 ) as endogenous controls. All reactions had a final cDNA concentration of 1 ng μl −1 and a primer concentration of 200 mM. The reactions were run on a StepOnePlusTM Real-Time PCR system (Applied Biosystems) using the SYBR Green master mix (Roche, Switzerland) with an annealing temperature of 58 °C and following the manufacturer’s protocols. Primers were designed with the software GenScript Real-Time PCR (Taqman) Primer Design available at https://www.genscript.com/ssl-bin/app/primer . All primers were designed to span over exons to avoid gDNA contamination (see Supplementary Table 3 for details). Primer efficiencies of the experimental primers ( fhl2a and fhl2b ) were comparable to the efficiency of the endogenous controls rpl7 and rpsa3 . We conducted the following experiments: qPCR experiment 1: Egg-spots were separated from the anal fin tissue in six male A. burtoni and five male C. pulpican . Relative quantity values were calculated for each sample, and the differential expression between anal fin (reference) and egg-spot tissue was analysed with a paired t -test using GraphPad Prism version 5.0a for Mac OS X ( www.graphpad.com ). qPCR experiment 2: fhl2a, fhl2b, csf1ra, mitfa, pnp4a and csf1b expression was measured in RNA extracted from A. burtoni fins at four different developmental stages [22] . Here, csf1ra was included as xanthophore marker [16] , mitfa and pnp4a as melanophore and iridophore markers [51] , respectively, and csf1b because of its role in pigment pattern organization in zebrafish [29] , [30] . We used three biological replicates for each developmental stage, and each replicate consisted of a sample pool of three fins, except for the youngest stage at 15 mm, where we pooled five fins. The first developmental stage was used as reference tissue. qPCR experiment 3: fhl2a and fhl2b expression was measured in RNA extracted from different tissues from three males from C. pulpican and N. crassus (gills, liver, testis, brain, heart, eye, skin, muscle, oral jaw, pharyngeal jaw and egg-spot). Although N. crassus does not have egg-spots, we separated its anal fin into an area corresponding to egg-spots in haplochromines and a section corresponding to anal fin tissue (the ‘egg-spot’ region was defined according to the egg-spot positioning in A. burtoni ). Expression was compared among tissues for each species using gills as reference tissue. The same experiment was performed for D. rerio and O. latipes (two teleost outgroups), using ef1a and rpl13a (ref. 52 ), as well as rpl7 and 18sRNA (ref. 53 ) as endogenous controls, respectively. Cloning of fhl2a and fhl2b and RNA in situ hybridization A. burtoni fhl2a and fhl2b coding fragments were amplified by PCR (for primer information, see Supplementary Table 3 ) using Phusion Master Mix with High Fidelity buffer (New England BioLabs, USA) following the manufacturer’s guidelines. These fragments were cloned into pCR4-TOPO TA vector using the TOPO TA cloning kit (Invitrogen). Plasmid extractions were done with GenElute Plasmid Miniprep Kit (Sigma-Aldrich). RNA probes were synthetized with the DIG RNA labelling kit (SP6/T7) (Roche). The insertion and direction of the fragments was confirmed by Sanger sequencing using M13 primers (available with the cloning kit) and BigDye terminator reaction chemistry (Applied Biosystems) on an AB3130 xl Genetic Analyzer (Applied Biosystems). In situ hybridization was performed in 12 fins from A. burtoni males, six for fhl2a and six for fhl2b . The protocol was executed as described in ref. 16 , except for an intermediate proteinase K treatment (20 min at a final concentration of 15 μg ml −1 ) and for the hybridization temperature (65 °C). Synteny analysis of teleost fhl2 paralogs The Synteny Database ( http://syntenydb.uoregon.edu [54] ) was used to generate dotplots of the human FHL2 gene (ENSG00000115641) region on chromosome Hsa2 and the genomes of medaka ( Supplementary Fig. 2a ) and zebrafish ( Supplementary Fig. 2b ). Double-conserved synteny between the human FHL2 gene and the fhl2a and fhl2b paralogons in teleost genomes provide evidence that the teleost fhl2 paralogs were generated during the teleost genome duplication. fhl2a/fhl2b coding region sequencing and analysis We then used cDNA pools extracted from anal fin tissue to amplify and sequence the coding region of fhl2a and fhl2b in a phylogenetically representative set of 26 cichlid species (21 Tanganyikan species, three species from Lake Malawi and two species from the Lake Victoria basin). This taxon sampling included 14 species belonging to the haplochromines and 12 species belonging to other East African cichlid tribes not featuring the egg-spot trait ( Supplementary Table 4 ). fhl2a and fhl2b coding regions were fully sequenced (from start to stop codon) in five individuals per species in order to evaluate the rate of molecular evolution among cichlids. For PCR amplification, we used Phusion Master Mix and cichlid-specific primers (for primer information, see Supplementary Table 3 ) designed with Primer3 (ref. 55 ). PCR products were visualized with electrophoresis in a 1.5% agarose gel using GelRed (Biotium, USA). In cases where multiple bands were present, we purified the correct size fragment from the gel using the GenElute Gel Extraction Kit (Sigma-Aldrich). PCR products were enzymatically cleaned with ExoSAP-IT (Affymetrix, USA) and sequenced with BigDye 3.1 Ready reaction mix (Applied Biosystems)—after BigDye XTerminator purificaton (Applied Biosystems)—on an AB3130 xl Genetic Analyzer. Sequences were corrected, trimmed and aligned manually in CODONCODE ALIGNER (CodonCode Corporation). fhl2 phylogenetic analysis fhl2a and fhl2b sequences from non-cichlid teleosts and fhl2 sequences from tetrapods were retrieved from ENSEMBL [56] (species names, gene names and accession numbers are available in Supplementary Table 5 ). We then constructed gene trees based on these sequences and on a subset of the cichlid sequences obtained in the previous step (information available in Supplementary Table 4 ) in order to confirm the orthologous and paralogous relationships of both duplicates. Sequences were aligned with CLUSTALW2 ( ref. 57 ) using default parameters. The most appropriate model of sequence evolution was determined with JMODELTEST as described above. Phylogenetic analyses were performed with MRBAYES (1 million generations; 25% burn-in). Tests for positive selection in fhl2a and fhl2b Using PAUP* 4.0b10 (ref. 58 ), we first compiled a maximum likelihood tree based on the mitochondrial ND2 gene, including all species used for the positive selection analyses (see Supplementary Table 6 for species and GenBank accession numbers). We used the GTR+Γ model with base frequencies and substitution rate matrix estimated from the data (as suggested by JMODELTEST [42] ). We then ran CODEML implemented in PAML version 4.4b to test for branch-specific adaptive evolution in fhl2a and fhl2b applying the branch-site model (free-ratios model with ω allowed to vary) [59] , [60] . The branch comparisons and results are shown in Supplementary Table 7 . Identification of CNEs We then made use of the five available cichlid genomes [61] to identify CNEs that could explain the difference in expression of fhl2a and fhl2b between haplochromines and non-haplochromines (note that there are three haplochromine genomes available: A. burtoni, Pu. nyererei, M. zebra ; and two genomes belonging to more ancestral cichlid lineages: N. brichardi and Or. niloticus ). For this analysis, we also included the respective genomic regions of four other teleost species ( O. latipes , Ta. rubripes , Te. nigroviridis and G. aculeatus ). More specifically, we extracted the genomic scaffolds containing fhl2a and fhl2b from the available cichlid genomes using BLAST v. 2.2.25 and the BIOCONDUCTOR R package BIOSTRINGS [62] to extract 5–6 kb of sequence containing fhl2a and fhl2b from these scaffolds. Comparative analyses of the fhl2a and fhl2b genomic regions were done with MVISTA (genome.lbl.gov/vista) [63] using the LAGAN alignment tool [64] ; A. burtoni was used as a reference for the alignment. We applied the repeat masking option with Ta. rubripes (Fugu) as reference. CNEs were defined as any non-coding section longer than 100 bp that showed at least 70% sequence identity with A. burtoni . Sequencing of the upstream region of fhl2b In order to confirm whether the AFC-SINE insertion was specific to egg-spot bearing haplochromines, we amplified the genomic region upstream of the fhl2b open reading frame in 19 additional cichlid species (10 haplochromines and 9 non-haplochromines). PCR amplification was performed as described above. For sequencing, we used four different primers, the two used in the amplification reaction and two internal primers, one haplochromine specific and another non-haplochromine specific. For detailed information about species and primers, see Supplementary Table 8 . Alignment of AFC-SINES from the A. burtoni genome SINE elements were identified using the SINE insertion sequence 5′ of the fhl2b gene of A. burtoni as query in a local BLASTn search [49] with default settings against the A. burtoni reference genome. Blast hits were retrieved using custom scripts and extended to a region of 200-bp upstream and downstream of the identified sequence. Sequences were aligned using MAFFT v. 6 (ref. 41 ) with default settings and allowing for adjustment of sequence direction according to the reference sequence. The alignment was loaded into CODONCODE ALIGNER for manual correction and end trimming. Sequences shorter than 50 bp were excluded from the alignment. The final alignment contained 407 sequences that were used to build the A. burtoni SINE consensus sequence using the consensus method implemented in CODONCODE ALIGNER with a percentage-based consensus and a cutoff of 25%. The AFC-SINE element in the fhl2b promoter region was compared with the consensus sequence and available full-length AFC-SINE elements of cichlids in order to determine whether it was an insertion or deletion in haplochromines ( Supplementary Table 8 ). Characterization of fhl2b upstream genomic region in cichlids The fhl2b genomic regions of the five cichlid genomes ( A. burtoni , M. zebra , Pu. nyererei , N. brichardi , and O. niloticus ) were loaded into CODONCODE ALIGNER and assembled (large gap alignments settings, identity cutoff 70%). Assemblies were manually corrected. Transposable element sequences were identified using the Repeat Masking function of REPBASE UNIT ( http://www.girinst.org/censor/index.php ) against all sequence sources and the bl2seq function of BLASTn [49] . Supplementary Fig. 6 shows a scheme of the transposable element composition of this genomic region in several cichlid species. CNEs construct cloning and injection in zebrafish We designed three genetic constructs containing the AFC-SINE and intron 1 of fhl2b of three cichlid species ( A. burtoni , P. philander and N. sexfasciatus ) ( Fig. 4 ) and one containing the 5′-untranslated region, exon 1 and intron 1 of A. burtoni fhl2a . The three fragments were amplified with PCR as described above (see Supplementary Table 3 for primer information). All fragments were cloned into a pCR8/GW/TOPO vector (Invitrogen) following the manufacturer’s specifications. Sequence identity and direction of fragment insertion were confirmed via Sanger sequencing (as described above) using M13 primers. All plasmid extractions were performed with GenElute Plasmid Miniprep Kit (Sigma-Aldrich). We then recombined these fragments into the Zebrafish Enhancer Detection ZED vector [65] following the protocol specified in ref. 66 . Recombination into the ZED plasmid was performed taking into consideration the original orientation of the fhl2b genomic region. The resulting ZED plasmids were then purified with the DNA clean and concentrator −5 Kit (Zymo Research, USA). Injections were performed with 1 nl into one-/two-cell stage zebrafish ( D. rerio ) embryos ( A. burtoni construct was injected in wild-type strains AB and ABxEK, P. philander and N. sexfasciatus constructs were injected in wild-type strain ABxEK) with 25 ng μl −1 plasmid and 35 ng μl −1 Tol2 transposase mRNA. By outcrossing to wild-type zebrafish, we created five F2 stable transgenic lines for the A. burtoni construct, two F1 stable transgenic lines for the P. philander construct, and finally one F1 stable transgenic line for the N. sexfasciatus construct. Fish were raised and kept according to standard procedures [67] . Zebrafish were imaged using a Leica point scanning confocal microscope SP5-II-matrix and Zeiss LSM5 Pascal confocal microscope. Fixation and dehydration of cichlid fins In order to determine the pigment cell composition of egg-spots (and especially whether they contain iridophores in addition to xanthophores), we dissected A. burtoni anal fins. To better understand the morphological differences between non-haplochromine and haplochromine fins, we further dissected three N. crassus anal fins. To visualize iridophores, we removed the pteridine pigments of the overlying xanthophores by fixating the fin in 4% paraformaldehyde–PBS for 1 h at room temperature and washing it in a series of methanol:PBS dilutions (25%, 50%, 75% and 100%). Pictures were taken after 6 days in 100% methanol at −20 °C. How to cite this article: Santos, M. E. et al . The evolution of cichlid fish egg-spots is linked with a cis -regulatory change. Nat. Commun. 5:5149 doi: 10.1038/ncomms6149 (2014). Accession codes : All nucleotide sequences reported in this study have been deposited in GenBank/EMBL/DDBJ under the accession codes KM263618 to KM264016 . All the short reads have been deposited in GenBank/EMBL/DDBJ Sequence Read Archive (SRA) under the BioProject ID PRJNA25755 .